Concentration memory-dependent synaptic plasticity of a taste circuit regulates salt concentration chemotaxis inCaenorhabditis elegans It is poorly understood how sensory systems memorize the intensity of sensory stimulus, compare it with a newly sensed stimulus, and regulate the orientation behaviour based on the memory. Here we report that Caenorhabditis elegans memorizes the environmental salt concentration during cultivation and exhibits a strong behavioural preference for this concentration. The right-sided amphid gustatory neuron known as ASER, senses decreases in salt concentration, and this information is transmitted to the postsynaptic AIB interneurons only in the salt concentration range lower than the cultivation concentration. In this range, animals migrate towards higher concentration by promoting turning behaviour upon decreases in salt concentration. These observations provide a mechanism for adjusting the orientation behaviour based on the memory of sensory stimulus using a simple neural circuit. All living animals are endowed with the capacity to seek optimal ambient conditions. Such behaviour requires memorizing the intensity of sensory stimulus associated with favourable conditions, recognizing the spatio-temporal changes of the stimulus intensity under current conditions, comparing it with the memorized stimulus intensity and regulating the motor output to generate a movement towards a preferred direction. However, in most sensory systems how stimulus intensity is memorized and how distinct orientation behaviours are generated depending on the memory have been poorly explored. Sodium chloride was identified as a chemoattractant for C. elegans [1] . Based on this view the mechanisms of salt chemotaxis has been examined for decades. Amphid taste neurons ASE, which consist of two morphologically symmetric neurons on the left (ASEL) and the right (ASER), have a predominant role in chemotaxis to NaCl and other inorganic salts [2] , [3] , [4] . Calcium imaging experiments showed that these neurons are functionally asymmetric: ASER is depolarized by decreases in salt concentration, while ASEL responds to increases [5] . As activation of ASER and ASEL promotes redirecting turns and forward locomotion, respectively, it was suggested that the right and the left neurons have distinct roles but act in concert for migrating up salt gradient [5] . Through another line of studies on the migration behaviours, two distinct behavioural mechanisms that drive animals towards higher salt concentration have been characterized so far (see below) [6] , [7] . Despite these sets of knowledge, the physiological and mechanistic properties of the information flow for salt chemotaxis downstream of the sensory neurons have not been obvious, as ASEL and ASER form synapses onto overlapping targets ( Fig. 1a ). 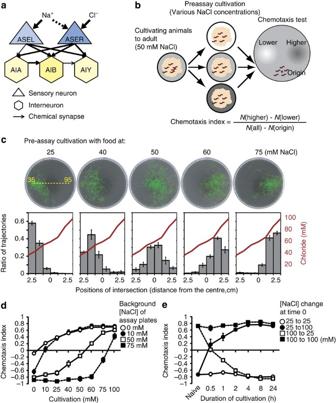Figure 1:C. elegansis attracted to the cultivation salt concentration. (a) A diagram of ASE salt-sensing neurons and downstream interneurons. Bold arrows indicate connections with more than five synapses19. (b) Procedure for the salt chemotaxis assay used in this study.Nindicates the number of animals within the region indicated in parentheses. (c) Representative trajectories of wild-type animals cultivated at different NaCl concentrations and tested on the plates with a NaCl gradient from 35 to 95 mM. Graphs show the positions of intersection between trajectories and the ridge of salt gradient (yellow dashed line). Mean±s.e.m.;n=4 assays. (d) Chemotaxis of wild type on the test plates similar to that inb, right, with different background NaCl concentrations. Salt gradients were generated with agar blocks that contained 150 mM (for higher concentration) and 0 mM (for lower concentration) of NaCl, which had not been changed from those used inc(see Methods for details). Mean±s.e.m.;n=6 assays. (e) Changes of preferred cultivation concentration. Wild-type animals were cultivated at either 25 or 100 mM of NaCl and transferred to 100 mM or 25 mM, reciprocally, or kept at the same concentration. Chemotaxis assays were performed at indicated time points using standard test plates as inc. ‘naive’ represents animals before transfer. Mean±s.e.m.;n=4 assays. Figure 1: C. elegans is attracted to the cultivation salt concentration. ( a ) A diagram of ASE salt-sensing neurons and downstream interneurons. Bold arrows indicate connections with more than five synapses [19] . ( b ) Procedure for the salt chemotaxis assay used in this study. N indicates the number of animals within the region indicated in parentheses. ( c ) Representative trajectories of wild-type animals cultivated at different NaCl concentrations and tested on the plates with a NaCl gradient from 35 to 95 mM. Graphs show the positions of intersection between trajectories and the ridge of salt gradient (yellow dashed line). Mean±s.e.m. ; n =4 assays. ( d ) Chemotaxis of wild type on the test plates similar to that in b , right, with different background NaCl concentrations. Salt gradients were generated with agar blocks that contained 150 mM (for higher concentration) and 0 mM (for lower concentration) of NaCl, which had not been changed from those used in c (see Methods for details). Mean±s.e.m. ; n =6 assays. ( e ) Changes of preferred cultivation concentration. Wild-type animals were cultivated at either 25 or 100 mM of NaCl and transferred to 100 mM or 25 mM, reciprocally, or kept at the same concentration. Chemotaxis assays were performed at indicated time points using standard test plates as in c . ‘naive’ represents animals before transfer. Mean±s.e.m. ; n =4 assays. Full size image Meanwhile, we have previously shown that pairing starvation with exposure to NaCl causes salt avoidance learning in C. elegans [8] . The insulin signalling pathway components, DAF-2 insulin receptor, AGE-1 phosphoinositide 3-kinase and AKT-1 AKT kinase, are required in ASER for this learning [9] . Activation of the Gq/DAG/PKC signalling pathway consisting of EGL-30 Gq, diacylglycerol (DAG) and PKC-1 (also known as TTX-4), a protein kinase C-ε isoform thought to act downstream of Gq, antagonizes the insulin signalling and promotes attraction to salt [10] . A similar starvation-dependent modulation of salt chemotaxis called gustatory plasticity has also been reported [11] . In this behaviour, ASH neurons, a pair of polymodal sensory neurons that drive avoidance of high osmolarity [12] , [13] , have a role in avoidance of salt [11] , [14] . Thus, chemotaxis to salt in C. elegans can be altered by previous experience of starvation. Here we provide evidence that chemotaxis to NaCl of well-fed animals is also a learned behaviour in C. elegans . Well-fed animals migrate up and down salt gradient towards the concentration of previous cultivation. A neural mechanism that generates experience-dependent switching of migration bias is provided. C. elegans attraction to NaCl cultivation concentration To observe preferred salt concentrations of C. elegans , we developed a behavioural assay in which adult animals are cultivated under defined concentrations of NaCl and their behaviour is subsequently examined on a NaCl gradient over a broad concentration range, typically spanning from 35 to 95 mM ( Fig. 1b and Supplementary Fig. S1 ). We found that wild-type C. elegans migrates to the salt concentration at which it has been cultivated with ample food ( Fig. 1c,d , Supplementary Fig. S2 , and see Methods for details). Preference for a particular salt concentration is plastic and animals adapt to a novel concentration within a few hours ( Fig. 1e ). Interestingly, animals avoid the salt concentration, which they have experienced under starvation conditions ( Supplementary Fig. S3a–c ). Thus, salt chemotaxis of C. elegans is affected by both the salt concentrations of preassay cultivation ( C cult ) and current environment on the test plate ( C test ). Fed animals move up salt gradient when C cult > C test and down the gradient when C cult < C test ; this relationship is reversed in starved animals. Migration to lower concentrations is unlikely to be an osmotic avoidance behaviour because the salt concentrations used in this study are much lower than those that evoke osmotic avoidance [11] , addition of osmolytes into the cultivation plates in place of NaCl does not affect chemotaxis to NaCl ( Supplementary Fig. S4a ), and chemotaxis to C cult is retained in mutants defective in osmotic response, osm-9 and osm-10 (a TRPV (transient receptor potential vanilloid) channel and a novel protein conserved in Caenorhabditis species, respectively, both required for osmosensory signalling in ASH neurons) ( Supplementary Fig. S4b ). In addition, the behavioural change is not due to a nonspecific effect on chemosensation or overall motility because chemotaxis to odorants was not affected by C cult ( Supplementary Fig. S5 ). Turning bias is regulated by salt concentration history Two behavioural strategies are known to regulate locomotion of C. elegans during salt chemotaxis. The first is klinokinesis, also called the pirouette strategy, in which migration is governed by biased random walk [6] . In this mechanism, the frequency of redirecting turns, or pirouettes, increases when the time derivative of salt concentration is negative, whereas locomotion towards higher concentrations is sustained by suppression of turns ( Fig. 2a , left). The second mechanism is klinotaxis, also called the weathervane mechanism, in which animals slowly curve towards preferred directions ( Fig. 2a , right) [7] . Both of these mechanisms originally accounted for overall migration towards higher salt concentrations in standard chemotaxis formats. 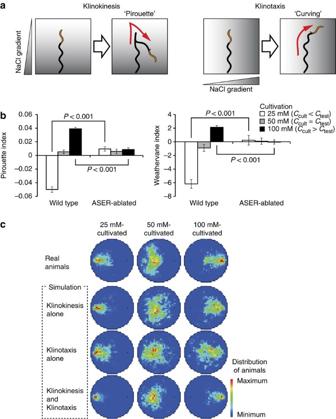Figure 2: Turning bias in klinokinesis and klinotaxis is regulated by relative salt concentrations betweenCcultandCtest. (a) Behavioural strategies of animals in chemotaxis: klinokinesis (left) and klinotaxis (right). (b) Bias of klinokinesis (left) and klinotaxis (right) represented by the pirouette index and the weathervane index, respectively. Positive indices indicate migration bias towards higher salt concentrations and negative indices indicate migration towards lower concentrations. Results of wild-type and ASER-ablated animals.n≥9 assays; Two-tailedt-test. (c) Probability of animal’s distribution during 250–500 s of chemotaxis tests. Top row, results from real animals; second row, simulation based solely on klinokinesis mechanism; third row, simulation based solely on klinotaxis mechanism; bottom row, simulation based on both mechanisms. Left column, results of animals cultivated at 25 mM NaCl; centre column, 50 mM; right column, 100 mM. Figure 2: Turning bias in klinokinesis and klinotaxis is regulated by relative salt concentrations between C cult and C test . ( a ) Behavioural strategies of animals in chemotaxis: klinokinesis (left) and klinotaxis (right). ( b ) Bias of klinokinesis (left) and klinotaxis (right) represented by the pirouette index and the weathervane index, respectively. Positive indices indicate migration bias towards higher salt concentrations and negative indices indicate migration towards lower concentrations. Results of wild-type and ASER-ablated animals. n ≥9 assays; Two-tailed t -test. ( c ) Probability of animal’s distribution during 250–500 s of chemotaxis tests. Top row, results from real animals; second row, simulation based solely on klinokinesis mechanism; third row, simulation based solely on klinotaxis mechanism; bottom row, simulation based on both mechanisms. Left column, results of animals cultivated at 25 mM NaCl; centre column, 50 mM; right column, 100 mM. Full size image Based on our observations that C. elegans can in fact migrate towards higher or lower salt concentrations depending on the relationship between C cult and C test , we quantitatively analysed the animals' behaviour and asked how chemotaxis to C cult is regulated by these two mechanisms, or by a novel mechanism such as orthotaxis, in which the velocity of animals is regulated by stimulus intensity [15] . When cultivation salt concentration was higher than test concentration ( C cult > C test ), klinokinesis was biased to drive migration towards higher concentrations: animals showed higher pirouette frequency if salt concentration decreased (d C /d t <0), but they showed lower pirouette frequency if salt concentration increased (d C /d t >0). On the other hand, when C cult < C test , the bias of klinokinesis was reversed ( Fig. 2b and Supplementary Fig. S6a , left panels). Reversal of behavioural strategy was also found in klinotaxis. Animals showed a positive klinotaxis when C cult > C test and negative klinotaxis when C cult < C test ( Fig. 2b and Supplementary Fig. S6a , right panels). When C cult = C test , there was no bias in klinokinesis but weakly negative klinotaxis was observed ( Fig. 2b and Supplementary Fig. S6a ). There was no obvious change in locomotion speed along with salt concentration regardless of C cult ( Supplementary Fig. S6d ), suggesting that contribution of orthotaxis is minimal, if any, in the current chemotaxis assay. Computer simulation based on these relationships showed that klinokinesis had a larger effect than klinotaxis in this assay while the behaviour is best reproduced with both mechanisms acting together ( Fig. 2c ). These results indicate that fed animals migrate towards both higher and lower concentrations by reversing motor output depending on relative salt concentrations between C cult and C test . Starvation also changes the properties of klinokinesis and klinotaxis. Klinokinesis bias was roughly reversed after 6 h of starvation ( Supplementary Figs. S3d and S6b ). Therefore, the bias changed depending on relative salt concentrations between C cult and C test , but in the opposite directions compared with fed conditions. The bias of klinotaxis was severely reduced but not reversed after starvation ( Supplementary Figs S3d and S6b ). These results are qualitatively similar to the previous observation on starvation-dependent salt avoidance [7] , with some minor differences probably due to the differences in test conditions. A pivotal role of ASER in concentration-dependent chemotaxis We asked which neurons are responsible for the behaviour ( Fig. 3a ). Loss of che-1 transcription factor, which is required for differentiation of ASE neurons [16] , caused a full loss of chemotaxis to C cult . Functional inactivation or genetic ablation of ASER [4] resulted in weak positive attraction to salt in which C cult -dependent plasticity is lost ( gcy-22 and ASER(-) in Fig. 3a ). In accordance with this, the bias of klinokinesis was slightly positive at any cultivation concentration, while klinotaxis bias was completely lost in ASER-ablated animals ( Fig. 2b and Supplementary Fig. S6c ). On the other hand, ablation of ASEL weakened the behavioural bias, but the animals still migrated up and down salt gradient (ASEL(-) in Fig. 3a ). These results demonstrate that ASER is most important for both migrating up and down salt gradient towards C cult . 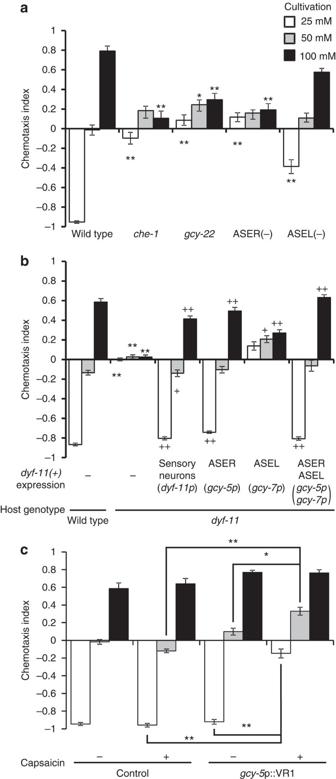Figure 3: ASER directs migration towards preferred salt concentrations. (a) Chemotaxis of ASE mutants. ASER is unresponsive to salt in the mutants of ASER-expressed guanylyl cyclasegcy-22(ref.4). See the main text for other strains. Mean±s.e.m.;n≥6 assays; (*)P<0.01, (**)P<0.001, different from wild-type cultivated at the same condition; Dunnett test. (b) Chemotaxis ofdyf-11and its cell-specific rescue lines. Mean±s.e.m.;n=10 assays; (**)P<0.001, different from wild type by two-tailedt-test; (+)P<0.01, (++)P<0.001, different fromdyf-11control by Dunnett test. (c) Aberrant stimulation of ASER alters preferred salt concentration. Chemotaxis tests were performed with or without 5 μM capsaicin included in the test plates. Mean±s.e.m.;n≥6 assays; (*)P<0.01, (**)P<0.001; Tukey test. Figure 3: ASER directs migration towards preferred salt concentrations. ( a ) Chemotaxis of ASE mutants. ASER is unresponsive to salt in the mutants of ASER-expressed guanylyl cyclase gcy-22 (ref. 4 ). See the main text for other strains. Mean±s.e.m. ; n ≥6 assays; (*) P <0.01, (**) P <0.001, different from wild-type cultivated at the same condition; Dunnett test. ( b ) Chemotaxis of dyf-11 and its cell-specific rescue lines. Mean±s.e.m. ; n =10 assays; (**) P <0.001, different from wild type by two-tailed t -test; (+) P <0.01, (++) P <0.001, different from dyf-11 control by Dunnett test. ( c ) Aberrant stimulation of ASER alters preferred salt concentration. Chemotaxis tests were performed with or without 5 μM capsaicin included in the test plates. Mean±s.e.m. ; n ≥6 assays; (*) P <0.01, (**) P <0.001; Tukey test. Full size image We next examined whether ASER is sufficient for the behaviour by cell-specific recovery of sensory input ( Fig. 3b ). dyf-11 encodes a component of ciliary transport, and due to the absence of sensory cilia, the dyf-11 mutants are severely impaired in sensing chemicals [17] . Cell-specific expression of dyf-11 complementary DNA (cDNA) in ASER fully rescued chemotaxis to C cult . Collectively, we conclude that input to ASER is necessary and sufficient for the behaviour: a single sensory neuron ASER can instruct the animal’s migration both up and down salt gradient. If ASER neuron alone can drive the chemotaxis to C cult , modulating the activity of ASER should shift the salt concentration preference. In fact, sustained activation of ASER during chemotaxis assay by TRPV1 (transient receptor potential vanilloid receptor 1, also known as VR1), a mammalian cation channel opened by capsaicin [5] , [18] , changed the preferred salt concentration of the animals towards higher salt concentrations ( Fig. 3c ). Synaptic plasticity occurs between ASER and AIB How can ASER and its downstream neural circuit encode memorized salt concentrations and generate bidirectional behaviour depending on previous experience? We addressed this question by examining whether the responses of these neurons change depending on C cult , through monitoring the intracellular calcium dynamics using the calcium indicator G-CaMP [18] . Responses of ASER to salt concentration change from 50 to 25 mM were larger in animals cultivated at higher salt concentrations, in the range of C cult between 0 and 50 mM, but the magnitude of the responses saturated at higher C cult ( Fig. 4a and Supplementary Table S1 ). We next examined the responses of AIB interneurons, which are directly innervated by ASER ( Fig. 1a ) [19] . We have recently found that AIB neurons are activated by reduction of salt concentration and the response is diminished after prolonged exposure to salt under starvation [18] . In the current assay, a NaCl down-step from 50 to 25 mM activated AIB after cultivation at 50 mM or higher, but not after cultivation at 25 mM or lower ( Fig. 4b ). These results, along with experiments using different stimulus concentrations ( Supplementary Fig. S7 and Supplementary Table S1 ), indicated that the magnitude of calcium response is modulated by the salt experience in both ASER and AIB. ASER showed graded responses according to the C cult . Exceptions were the cases in which NaCl was completely removed (from 25 to 0 mM) and those noted above ( C cult ≥50 mM in Fig. 4a ). Under these conditions, the fluorescence intensity might not be proportional to cellular responses. On the other hand, AIB responded prominently when C cult was higher than stimulus concentration, but they did not respond when C cult was lower than stimulus concentration. This neuronal response parallels the behaviour: animals respond to decreases in salt concentration by increased turning only when C cult > C test ( Supplementary Fig. S6a ). 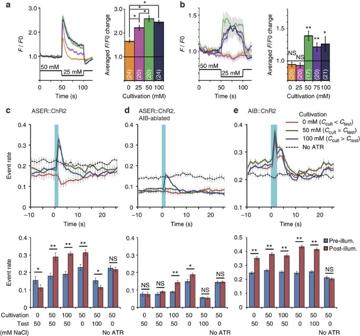Figure 4: Concentration-dependent behavioural plasticity occurs between ASER and AIB. (a,b) Calcium responses of ASER (a) and AIB (b) of wild-type animals to a NaCl down-step from 50 to 25 mM (traces). Averaged fluorescence changes during 5 s (ASER) or 25 s (AIB) after stimulation (bar graphs). Shaded region around the response curve and the error bars represents s.e.m. The number of tested animals for each condition is indicated in parentheses. Statistics for ASER responses in panelaare: (*)P<0.01; Tukey test; details are shown inSupplementary Table S1. Statistics for AIB responses in panelbare: (*)P<0.01, (**)P<0.001, (NS) not significant; Mann–WhitneyU-test compared with prestimulation. (c–e) Turning behaviours evoked by optical stimulation of ASER (c,d) or AIB (e) by ChR2. AIB interneurons are ablated ind. Animals were cultivated at the indicated conditions and illuminated by blue light (blue vertical lines) on agar plates with 50 mM NaCl (top). Bar graphs show averaged turning rate during pre- and post-illumination periods (bottom). Mean±s.e.m.;n≥6 assays; (*)P<0.01, (**)P<0.001, (NS) not significant; two-tailedt-test. Figure 4: Concentration-dependent behavioural plasticity occurs between ASER and AIB. ( a , b ) Calcium responses of ASER ( a ) and AIB ( b ) of wild-type animals to a NaCl down-step from 50 to 25 mM (traces). Averaged fluorescence changes during 5 s (ASER) or 25 s (AIB) after stimulation (bar graphs). Shaded region around the response curve and the error bars represents s.e.m. The number of tested animals for each condition is indicated in parentheses. Statistics for ASER responses in panel a are: (*) P <0.01; Tukey test; details are shown in Supplementary Table S1 . Statistics for AIB responses in panel b are: (*) P <0.01, (**) P <0.001, (NS) not significant; Mann–Whitney U -test compared with prestimulation. ( c – e ) Turning behaviours evoked by optical stimulation of ASER ( c , d ) or AIB ( e ) by ChR2. AIB interneurons are ablated in d . Animals were cultivated at the indicated conditions and illuminated by blue light (blue vertical lines) on agar plates with 50 mM NaCl (top). Bar graphs show averaged turning rate during pre- and post-illumination periods (bottom). Mean±s.e.m. ; n ≥6 assays; (*) P <0.01, (**) P <0.001, (NS) not significant; two-tailed t -test. Full size image AIB receives synaptic inputs from many sensory neurons, but we reasoned that the plasticity of neuronal responses is likely dependent on ASER because input from ASER is sufficient for chemotaxis to C cult . To test this, we performed calcium imaging of ASER and AIB in dyf-11 mutants, which have impaired sensory cilia. In dyf-11 mutants, stimulus-evoked calcium responses were small and the C cult -dependent plasticity was completely abolished in both ASER and AIB ( Supplementary Fig. S8a ). In the animals whose ASER was solely rescued, the response of ASER was fully restored. The initial calcium response of AIB was also restored to be comparable to that of wild type but it was not sustained, indicating that the sustained response requires inputs from neurons other than ASER. Importantly, the C cult -dependent plasticity of AIB response was essentially the same as wild type, demonstrating that the plasticity of AIB response depends on ASER ( Supplementary Fig. S8b ). Activation of AIB triggers reversals and turning [20] , [21] , and is likely to promote directional changes during chemotaxis [22] . To examine whether ASER- and AIB-evoked turning is actually modulated by salt-concentration experience, we took an optogenetic approach by expressing channelrhodopsin-2 (ChR2) in these neurons. ChR2 is a light-gated cation channel and its activation by light illumination depolarizes neurons [23] . Activation of ASER by ChR2 promoted turning when salt concentration of the cultivation plate was above that of the test plate ( C cult ≥ C test ), while it suppressed turning when C cult < C test ( Fig. 4c ). On the other hand, activation of AIB promoted turning irrespective of C cult ( Fig. 4e ). If AIB neurons mediate information from ASER, ablation of AIB may affect the probability of ASER-evoked turning. Loss of AIB resulted in overall decrease in pirouette frequency: the basal pirouette index of 50 mM NaCl-cultivated animals was 0.043±0.001 in wild-type and 0.022±0.001 in AIB-ablated animals ( n ≥16, mean±s.e.m., P <0.001 by two-tailed t -test, see Methods for details). When ASER was stimulated in AIB-ablated animals, ASER-evoked promotion of turning was still observed under C cult > C test conditions but the magnitude was smaller. On the other hand, changes of turning rate under the conditions of C cult = C test and C cult < C test were eliminated ( Fig. 4d ). These results indicate that the ASER-evoked change in turning probability is at least partly regulated through AIB and the synaptic connection between ASER and the downstream interneurons is one of the sites of modulation by salt-concentration experience. Quantitative behavioural analyses of AIB-ablated animals revealed that although AIB was apparently involved in regulation of pirouette frequency, klinotaxis was intact in AIB-ablated animals ( Supplementary Fig. S9a ). Besides, ablation of AIB barely affected chemotaxis in the current assay ( Supplementary Fig. S9b ). These results suggest that the information from ASER is transferred also by interneurons that act parallel to AIB in salt chemotaxis (see Discussion). As ASER alone can regulate the whole orientation behaviour on salt gradient ( Fig. 3b ), it is possible that ASER also mediates the behavioural response to increase in salt concentration. In accordance with this idea, the klinokinesis bias upon increase in salt concentrations is completely lost in ASER-ablated animals ( Supplementary Fig. S6c ). Salt-concentration increase de-activates ASER [5] . Stepwise increase in salt concentration actually resulted in a rapid decrease in G-CaMP fluorescence at the end of stimulation in our imaging experiments ( Fig. 4a ). However, the responses were less prominent when salt up-step was delivered after 8 min of incubation at a constant salt concentration ( Supplementary Fig. S7d ), which precluded further analyses on up-step responses (see Discussion). Gq/DAG/PKC signalling in ASER regulates migration bias To see whether the insulin signalling and the Gq/DAG/PKC signalling act in cultivation concentration-dependent chemotaxis plasticity, we examined salt chemotaxis of the mutants after cultivation under fed and starved conditions. Mutants of daf-2 , age-1 and akt-1 , as well as ins-1 , a putative ligand for DAF-2, were defective in avoidance of C cult after starvation. But attraction to C cult associated with food was less impaired in these mutants ( Fig. 5a ). These results indicate that the insulin pathway acts to switch the direction of salt chemotaxis after starvation. Activation of the Gq/DAG/PKC pathway by addition of a DAG analogue phorbol 12-myristate 13-acetate to the cultivation media or by a putative gain-of-function mutation in egl-30 (ref. 9 ) resulted in migration to higher salt concentrations regardless of food conditions ( Fig. 5c,d ). Conversely, inactivation of this pathway by a null mutation in pkc-1 caused migration to lower concentrations ( Fig. 5d ). Consistent with the central roles of ASER in the behaviour, cell-specific expression of an activated form of PKC-1 or inactivation of pkc-1 in ASER mimicked the mutations that activate or inactivate the pathway, respectively ( Fig. 5e ). Therefore, the Gq/DAG/PKC pathway in ASER may act to determine the migration bias on salt gradient under both fed and starved conditions. 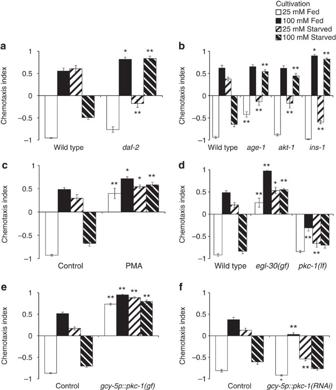Figure 5: Insulin signalling is involved in starvation-induced chemotaxis plasticity, whereas Gq/DAG/PKC signalling regulates migration bias. (a)daf-2(e1370)mutants show defects in starvation-dependent modulation of salt chemotaxis. As the mutants become dauer larvae at a high temperature, animals were grown to L4 at 15 °C, then transferred to 25 °C at which temperature preassay cultivation and chemotaxis tests were conducted. Mean±s.e.m.;n=6 assays; (*)P<0.01, (**)P<0.001, different from wild type cultivated at the same condition; two-tailedt-test. (b) Chemotaxis of other insulin pathway mutants. See the main text for description of the strains. Mean±s.e.m.;n≥6 assays; (*)P<0.01, (**)P<0.001, different from wild type cultivated at the same condition; Dunnett test. (c) Addition of 0.25 mg l−1phorbol 12-myristate 13-acetate (PMA) to cultivation media promotes salt attraction. Mean±s.e.m.;n=6 assays; (*)P<0.01, (**)P<0.001, different from control cultivated at the same condition; two-tailedt-test. (d) Chemotaxis ofegl-30(pe914)andpkc-1(nj3)mutants. See text for description of the strains. Mean±s.e.m.;n≥6 assays; (*)P<0.01, (**)P<0.001, different from wild type cultivated at the same condition; Dunnett test. (e) ASER-specific activation of PKC-1. Mean±s.e.m.;n=7 assays; (**)P<0.001, different from control cultivated at the same condition; two-tailedt-test. (f) ASER-specific inactivation ofpkc-1by cell-specific double-stranded RNA expression. Mean±s.e.m.;n=10 assays; (*)P<0.01, (**)P<0.001, different from control cultivated at the same condition; two-tailedt-test. Figure 5: Insulin signalling is involved in starvation-induced chemotaxis plasticity, whereas Gq/DAG/PKC signalling regulates migration bias. ( a ) daf-2(e1370) mutants show defects in starvation-dependent modulation of salt chemotaxis. As the mutants become dauer larvae at a high temperature, animals were grown to L4 at 15 °C, then transferred to 25 °C at which temperature preassay cultivation and chemotaxis tests were conducted. Mean±s.e.m. ; n =6 assays; (*) P <0.01, (**) P <0.001, different from wild type cultivated at the same condition; two-tailed t -test. ( b ) Chemotaxis of other insulin pathway mutants. See the main text for description of the strains. Mean±s.e.m. ; n ≥6 assays; (*) P <0.01, (**) P <0.001, different from wild type cultivated at the same condition; Dunnett test. ( c ) Addition of 0.25 mg l −1 phorbol 12-myristate 13-acetate (PMA) to cultivation media promotes salt attraction. Mean±s.e.m. ; n =6 assays; (*) P <0.01, (**) P <0.001, different from control cultivated at the same condition; two-tailed t -test. ( d ) Chemotaxis of egl-30(pe914) and pkc-1(nj3) mutants. See text for description of the strains. Mean±s.e.m. ; n ≥6 assays; (*) P <0.01, (**) P <0.001, different from wild type cultivated at the same condition; Dunnett test. ( e ) ASER-specific activation of PKC-1. Mean±s.e.m. ; n =7 assays; (**) P <0.001, different from control cultivated at the same condition; two-tailed t -test. ( f ) ASER-specific inactivation of pkc-1 by cell-specific double-stranded RNA expression. Mean±s.e.m. ; n =10 assays; (*) P <0.01, (**) P <0.001, different from control cultivated at the same condition; two-tailed t -test. Full size image In agreement with this idea, we found that mutations in the phospholipase C (PLC)-ε plc-1 alter salt-concentration preference ( Supplementary Fig. S10a and see Methods for details). A semi-dominant mutation plc-1(pe1237) and a reduction-of-function mutation plc-1(pe1238) showed opposite phenotypes: the preferred salt concentration was upshifted in pe1237 and downshifted in pe1238 ( Fig. 6a ). A transcriptional reporter of plc-1 was expressed in head sensory neurons AWC, AFD, ASE, ASG and BAG, as well as interneurons RIF, ventral nerve cord neurons, tail neurons and body muscles ( Supplementary Fig. S10b ). Cell-specific rescue experiments showed that PLC-1 acts in ASER but not in ASEL or the downstream interneurons including AIB ( Fig. 6b ). Calcium responses of ASER, including the modulation by C cult , was comparable to that of wild type in both plc-1(pe1237) and plc-1(pe1238) mutants, suggesting that DAG signalling may not affect salt sensing of ASER ( Fig. 6c,d ). In contrast, the responses of AIB were augmented in plc-1(pe1237) after cultivation at 0 mM ( Fig. 6c ), while diminished in plc-1(pe1238) after cultivation at 50 mM or higher ( Fig. 6d ). ASER-specific expression of plc-1(+) restored the responses of AIB in plc-1(pe1238) mutants without affecting the responses of ASER ( Fig. 6e ). Thus the property of AIB response well correlates with the altered behaviour in plc-1 mutants. These results are consistent with the idea that synaptic connection between ASER to the interneurons, which is modulated by salt experience of ASER, is the site of plasticity that underlies chemotaxis to preferred concentrations. Chemotaxis phenotype of the plc-1 mutants was weaker compared with the egl-30 Gq or pkc-1 nPKC mutants, which may be either because we used weak mutants of plc-1 (null mutants of plc-1 are lethal [24] ) or because another PLC, such as egl-8 , acts in parallel with plc-1 . 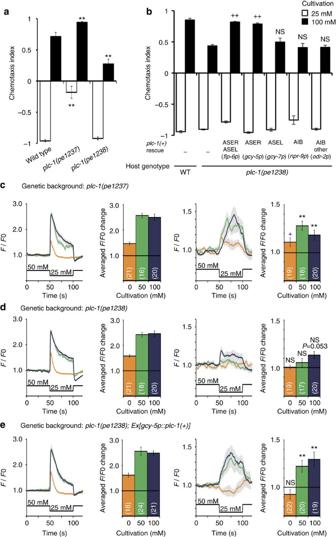Figure 6:plc-1is involved in chemotaxis and acts in ASER to modulate synaptic plasticity between ASER and AIB. (a) Salt chemotaxis ofplc-1mutants. See text for description of the mutants. Mean±s.e.m.;n=6 assays; (**)P<0.001, different from wild type; Dunnett test. (b) Chemotaxis of cell-specific rescue lines ofplc-1(pe1238). Mean±s.e.m.;n≥6 assays; (++)P<0.001, (NS) not significant, different fromplc-1(pe1238)control; Dunnett test. (c–e) Calcium responses of ASER (left panels) and AIB (right panels) inplc-1(pe1237)(c),plc-1(pe1238)(d) andplc-1(pe1238)animals whose ASER was solely rescued byplc-1cDNA (e). Averaged fluorescence changes during 5 s (ASER) or 25 s (AIB) after stimulation are shown in the bar graphs. Shaded region around the response curve and the error bars represents s.e.m. The number of tested animals for each condition is indicated in parentheses. Statistics for ASER responses are shown in Supplementary Table S1. Statistics for AIB responses are: (+)P<0.05, (**)P<0.001, (NS) not significant; Mann–WhitneyU-test compared with prestimulation for panelsc–e. Figure 6: plc-1 is involved in chemotaxis and acts in ASER to modulate synaptic plasticity between ASER and AIB. ( a ) Salt chemotaxis of plc-1 mutants. See text for description of the mutants. Mean±s.e.m. ; n =6 assays; (**) P <0.001, different from wild type; Dunnett test. ( b ) Chemotaxis of cell-specific rescue lines of plc-1(pe1238) . Mean±s.e.m. ; n ≥6 assays; (++) P <0.001, (NS) not significant, different from plc-1(pe1238) control; Dunnett test. ( c – e ) Calcium responses of ASER (left panels) and AIB (right panels) in plc-1(pe1237) ( c ), plc-1(pe1238) ( d ) and plc-1(pe1238) animals whose ASER was solely rescued by plc-1 cDNA ( e ). Averaged fluorescence changes during 5 s (ASER) or 25 s (AIB) after stimulation are shown in the bar graphs. Shaded region around the response curve and the error bars represents s.e.m. The number of tested animals for each condition is indicated in parentheses. Statistics for ASER responses are shown in Supplementary Table S1. Statistics for AIB responses are: (+) P <0.05, (**) P <0.001, (NS) not significant; Mann–Whitney U -test compared with prestimulation for panels c – e . Full size image Seeking of an acclimated environmental condition is commonly observed in adaptive behaviours in migrant animals. Here we showed that C. elegans migrates to the salt concentration at which it has previously been fed. Such a behavioural strategy might be beneficial for staying at food-rich environment or finding a new food source in the neighbourhood. After cultivation at higher concentrations ( C cult > C test ), decreases in salt concentration activates ASER and AIB and induces turning behaviour, whereby driving the animals to higher salt concentrations ( Supplementary Fig. S11 ), while when animals were cultivated at lower concentrations ( C cult < C test ), stimulation of ASER suppressed directional changes ( Fig. 4c ). As the ASER-evoked stimulation of turning in the C cult > C test conditions still occurred in AIB-ablated animals ( Fig. 4d ), information is mediated by uncharacterized neuron(s) innervated by ASER as well as AIB ( Supplementary Fig. S11 ). Furthermore, AIB is not required for klinotaxis in the current test conditions ( Supplementary Fig. S9a ). These observations indicate that processing of salt information does not rely on a single interneuron class but is processed by a parallel circuit as in olfaction or thermosensation in this organism [22] , [25] . ASER apparently senses not only decrease but also increase in salt concentrations as manifested by a decrease in intracellular calcium level [5] , and our behavioural analyses indicated that ASER is essential for behavioural response to increase, as well as decrease in salt concentrations ( Supplementary Fig. S6a,c ). However, we could not detect sufficient changes in the ASER calcium levels ( Supplementary Fig. S7d ), which precluded further analyses of the activities of neural circuits that are linked to the behaviour of animals migrating up the gradient. This could be due to the difference in calcium indicators because GCaMP2 used in the current study has a larger K d than YC2.12 used in the previous study [5] and therefore could be less sensitive to low levels of intracellular calcium. Further study is needed for clarifying the neural basis of this behaviour. There are striking similarities between chemotaxis and thermotaxis not only in the homoeostatic behavioural patterns [26] , [27] but also in the role of DAG signalling; genetic manipulations that increase or decrease DAG signalling in the AFD thermosensory neurons result in migration to lower or higher temperature, respectively [28] . DAG pathway was also implicated in acclimation to ambient temperature through modulating synaptic output of AFD [29] . In ventral cord motor neurons, DAG positively regulates synaptic release through PKC-1 and UNC-13 (refs 30 , 31 ). By analogy, neurotransmission between ASER and AIB may be regulated by this pathway. There also remains a possibility that a threshold in the responses of ASER switches excitatory and inhibitory transmission to postsynaptic interneurons as has been recently suggested between AFD and AIY [32] . Strains and culture C. elegans strains and transgenic lines used in this study are listed in Supplementary Table S2 . All mutant strains were outcrossed multiple times with N2. Animals were cultivated at 20 °C under standard conditions unless otherwise noted [33] . Fast-growing E. coli NA22 was used as a food source in behavioural tests to avoid starvation. OP50 was used for imaging experiments because animals cultivated with NA22 tended to exhibit high background fluorescence in the intestine. Differences in the bacterial strains do not affect cultivation salt concentration-dependent chemotaxis ( Supplementary Fig. S2 ). Standard genetics methods were used to generate strains by crosses [33] . Behavioural tests To evaluate animal’s behaviour on salt gradient, a modified chemotaxis assay was used in this study. Animals were handled with chemotaxis buffer (25 mM potassium phosphate (pH 6.0), 1 mM CaCl 2 , 1 mM MgSO 4 ) supplemented with 50 mM NaCl. Test plates were prepared as shown in Supplementary Fig. S1a . The background agar was 8.5 cm in diameter and 1.76 mm in thickness (10 ml solution was poured) and included 50 mM NaCl and 2% agar in chemotaxis buffer. On top of the plate, two cylindrical agar blocks (each 14.5 mm in diameter and 5.3 mm in thickness, including either 0 mM (lower side) or 150 mM (higher side) of NaCl and 2% agar in chemotaxis buffer and excised from an agar plate using a cork borer) were placed at the positions 3 cm from the centre of the plate in the opposite directions for 18 h at 20 °C and removed just before assay. This procedure created a concentric salt gradient on the test plate with highest concentration at the centre of the high-salt block, lowest concentration at the opposite side and background concentration around the centre. The actual concentrations of chloride ion were measured using a chloride electrode (Horiba). The background was typically 55–56 mM, 3–4 mM higher than calculated, probably due to the trace amount of chloride in agar ( http://www.bd.com/ds/productCenter/ ) and by desiccation. Animals were grown to adults on standard nematode growth medium (NGM), and then transferred to NGM plates with various concentrations of NaCl for preassay cultivation for 6 h. Fifty to two-hundred animals were washed out from the plates, placed at the start point on the test plates (2.5 cm off centre), and allowed to run for 45 min. One microliter each of 0.5 M NaN 3 was spotted to the peak of NaCl gradient and to the opposite position to trap animals. The number of animals within a 2-cm radius from the centre of each agar block was considered to be attracted and the number of animals within a 1-cm radius from the start point was ignored from the total number of animals to calculate chemotaxis index ( Fig. 1b ). The indices of 1.0 and −1.0 represent complete preferences for higher and lower concentrations, respectively, and the index of zero represents preference for the background concentration, equal distribution to both sides or a random distribution. In Fig. 1d , salt gradients were generated on the test plates that contained indicated background NaCl concentrations, using agar blocks whose NaCl concentrations were unchanged. In Fig. 1e , the duration of preassay cultivation was varied as indicated. In Fig. 3c , 5 μM capsaicin (Sigma) or solvent alone (0.1% ethanol) was added to the test plates. In Fig. 5c , 0.25 mg l −1 of PMA (Sigma) or solvent (0.01% ethanol) was added to preassay cultivation. In all behavioural tests, at least four trials were independently performed for each data point and the results were statistically validated as described in each figure. Chemotaxis assays for odourants ( Supplementary Fig. S5 ) were performed as described [34] . Dilutions of odourants in ethanol were 1:1,000 for diacetyl and benzaldehyde, and no dilution for 2-nonanone. Salt chemotaxis test in Supplementary Fig. S5 was performed as described [9] with preassay cultivation. Calcium imaging Animals that express G-CaMP in ASER or AIB in wild-type background are described previously [18] , [22] . The latter was a gift from C. Bargmann. We found no obvious defects in salt chemotaxis in these animals. Reporter strains that carry particular genetic background were generated by genetic crosses ( Supplementary Table S2 ). Imaging experiments were performed as described [35] with modifications. Briefly, animals were cultivated on standard NGM until young adult and further incubated overnight on NGM with various concentrations of NaCl and whose osmolarity was adjusted to 350 mOsm. Animals were then immobilized by a microfluidic device [36] and NaCl concentration steps were delivered to their nose tip by switching the solutions (25 mM potassium phosphate (pH 6.0), 1 mM CaCl 2 , 1 mM MgSO 4 , 0.02% gelatin, NaCl at the indicated concentrations and glycerol to adjust their osmolarity to 350 mOsm). Time-lapse images were acquired with a DMI-6000B microscope (Leica) equipped with an HCX-PL-APO 63x objective (NA, 1.40), L5 filter set (a combination of 480/40 nm band-path excitation filter and 505 nm dichromatic mirror, Leica), and ImagEM EM-CCD camera (Hamamatsu) at two frames per second. The initial frame of recordings (Time=0 in traces) was fixed as 8 min after removal of animals from cultivation plates throughout this paper because prolonged duration of prestimulus incubation considerably affected the magnitude and duration of the response. Individual animals were subjected to single recording and replaced for each experiment. Average fluorescence intensity of the cell body was calculated by correcting the position of region of interest by Track Objects function of Metamorph software (Molecular devices) followed by subtracting the average intensity of a background region. The average fluorescence in a 10-s window (typically, Time=4–14 s) was set as F 0 and the fluorescence intensity relative to F 0 ( F / F 0) were calculated for a series of images. For traces, F / F 0 was averaged for all animals at each time point. For graphs, averaged F / F 0 during 5 s (ASER) or 25 s (AIB) after stimulation were calculated. Analysis of locomotion The worm tracking system simultaneously identifies and tracks tens of animals on a test plate, and extracts behavioural parameters of each animal [37] . Chemotaxis tests were prepared as described above, but only 30–50 animals were placed at the start point to reduce the chance of collision of animals. Images of the whole test plate were acquired for 30 min at one frame per second. Probability of pirouette and curving rate were calculated as described [7] . Pirouette index was defined as the difference of probability of pirouette between negative d C /d T rank and positive d C /d T rank. Weathervane index was defined as the slope of the regression line in relationship between NaCl gradient in normal direction and the curving rate. These values were calculated for each test, and average and s.e.m. were shown in figures. Concentrations of NaCl on the test plate were calculated by three-dimensional Euler's method based on Fick's low adopting D =0.000013 (cm 2 s −1 ) as diffusion constant for NaCl ( Supplementary Fig. S1b ). This enabled us to analyse locomotion of animals on salt gradient precisely. In Supplementary Fig. S6 , pirouette frequency was calculated according to the time derivative of salt concentration by 0.1 mM s −1 bins. Curving rate was calculated according to the NaCl gradient in normal direction by 0.5 mM mm −1 bins. Bins with <20 data points were omitted from further analyses. Data from the initial 500 s were used to calculate the behavioural parameters because most of the animals migrated to C cult within the period. The trajectories of animals in Fig. 1c and Supplementary Fig. S3a were reconstructed by the tracking system by excluding those interrupted by collision of animals. Simulation of animals’ behaviour was performed as described [7] except that the curving rate (change of movement direction per unit length of progression, degree mm −1 ) of the animals followed a first-order autoregression, namely where k =0.933 is a decay constant determined from the data of real animals [7] , and is a Gaussian white noise whose s.d. was also determined from real measurements. Optogenetics All optical stimulation experiments were carried out in lite-1(ce314) mutants to eliminate intrinsic light response [38] . For ASER-specific stimulation, animals that harbour chromosome-integrated gcy-5 promoter-driven ChR2 transgene, Is[gcy-5p::ChR2::yfp] (90 ng μl −1 ), were used. For AIB-specific activation, animals that carry extra-chromosomal Ex[npr-9p::ChR2::yfp] (90 ng μl −1 ) were used. A cDNA clone for murine caspase-1 (ref. 37 ) was expressed by npr-9 promoter to ablate AIB neurons. In the resultant Is[npr-9p::casp1] strain, AIB neurons were absent in >90% of animals. Adults grown on standard NGM plates were further cultivated overnight under various concentrations of salt supplemented with 5 μM all-trans retinal (Sigma). Their behaviour was tested on a retinal-free chemotaxis plate without salt gradient. One- (for ASER) or two-second (for AIB) pulse of blue light (peak wavelength=470 nm; 190 W m −2 ) was delivered by a ring-shaped light-emitting diode light (CCS). Each animal was tested six times with a 120-s interval between each test. Locomotion was monitored by the worm tracking system. The event rate was calculated as the ratio of animals that are during pirouettes, turns or pauses at each time point. At least six independent experiments were performed for each condition. Characterization of plc-1 plc-1(pe1237) was isolated by a genetic screen as a mutation that confers preference for high concentrations of salt [35] . We assigned the mutation to a predicted gene frm-9 /F31B12.3, which encodes a 4.1 ezrin-radixin-moesin (FERM) domain-containing protein with unknown function (WormBase Release WS230) ( Supplementary Fig. S10a ). Then, we obtained a deletion allele of the gene pe1238 by ultraviolet/trimethylpsoralen mutagenesis. Interestingly, pe1238 showed chemotaxis phenotype opposite to the original mutation; it preferred lower concentrations if compared with wild type ( Fig. 6a ). In the course of rescue experiments, we noticed that gene prediction of frm-9 is incomplete because fosmids that cover the entire frm-9 region, WRM065aD07 and WRM0620c09 failed to complement pe1238 ( Supplementary Fig. S10a ). Extensive reverse transcription–PCR experiments revealed that there exists a 10.6-kbp cDNA that spans from frm-9 to plc-1 /F31B12.1 ( Supplementary Fig. S10a ). PLC-1 regulates epidermal morphogenesis in embryogenesis and also function in spermatheca to regulate ovulation through production of inositol 1,4,5-triphosphate [24] , [39] . plc-1(tm753) showed chemotaxis defects similar to that of pe1238 , as well as partial sterility consistent with the previous report [24] . The cDNA clone for long isoform, but not the short isoform of plc-1 , rescued the salt preference defects in plc-1(pe1238) ( Fig. 6b and Supplementary Fig. S10a ). These results collectively show that the newly identified isoform is required for salt chemotaxis. The amino terminal region of PLC-1 is not required for fertility and may function as a regulatory domain of the enzyme. Molecular biology Plasmids were generated by the GATEWAY system (Invitrogen) as described [34] . Details are available at our web site ( http://molecular-ethology.biochem.s.u-tokyo.ac.jp/Gateway/Gateway_overview1.html ) Promoters for flp-6 (ref. 40 ), odr-2 (ref. 41 ), dyf-11 (ref. 17 ), npr-9 (ref. 42 ), gcy-5 and gcy-7 (ref. 43 ) were described previously. Structure of the cDNA for plc-1 was determined by reverse transcription of total RNA of wild type followed by 5′- and 3′- rapid amplification of cDNA ends (RACE) using primers 5′-CCGTCTAGAACTAGTCCTCCTTTTTTTTTT-3′ for reverse transcription, 5′-TAGGTACCGGTTTAATTACCCAAGTTTGAG-3′ for 5′-RACE, and 5′-CCGTCTAGAACTAGTCCTCC-3′ for 3′-RACE. To generate a destination plasmid for plc-1 , full-length cDNA was amplified using primers 5′-GTGGACTCAATGCCAACATC-3′ and ATCACTCGTGTCTGGGATCCAT. A 5.1-kbp plc-1 promoter was amplified by PCR using primers 5′-ATGTCCTTACGCCAAGCATC-3′ and AAAATTTTCAGCATTTCAAACAT. Expression constructs for dyf-11 (ref. 17 ), pkc-1 (ref. 10 ) and fluorescence reporter proteins [44] were described previously. Transformation Germ-line transformations were performed by standard microinjection methods [45] . Expression constructs for dyf-11 were injected at 5 ng μl −1 along with transformation marker (20 ng μl −1 ) and pPD49.26 (75 ng μl −1 ) as carrier DNA. The expression constructs for plc-1 were introduced at 100 ng μl −1 with transformation marker (20 ng μl −1 ). An empty vector was introduced in place of the expression construct in control experiments. Cell-specific RNA interference Hairpin-structured double-stranded RNA for pkc-1 was expressed in a cell-specific manner using the pWormgate vector [46] . A 0.86 kb of pkc-1 cDNA fragment, which corresponds to the carboxyl terminal half of PKC-1, was driven by the gcy-5 promoter for ASER-specific expression. In control experiments, an empty pWormgate vector with gcy-5 promoter was introduced. Plasmids were introduced into wild-type animals at 100 ng μl −1 along with myo-3p::venus (15 ng μl −1 ). How to cite this article: Kunitomo, H. et al. Concentration memory-dependent synaptic plasticity of a taste circuit regulates salt concentration chemotaxis in Caenorhabditis elegans . Nat. Commun. 4:2210 doi: 10.1038/ncomms3210 (2013).